The sorting protein PACS-2 promotes ErbB signalling by regulating recycling of the metalloproteinase ADAM17 The metalloproteinase ADAM17 activates ErbB signalling by releasing ligands from the cell surface, a key step underlying epithelial development, growth and tumour progression. However, mechanisms acutely controlling ADAM17 cell-surface availability to modulate the extent of ErbB ligand release are poorly understood. Here, through a functional genome-wide siRNA screen, we identify the sorting protein PACS-2 as a regulator of ADAM17 trafficking and ErbB signalling. PACS-2 loss reduces ADAM17 cell-surface levels and ADAM17-dependent ErbB ligand shedding, without apparent effects on related proteases. PACS-2 co-localizes with ADAM17 on early endosomes and PACS-2 knockdown decreases the recycling and stability of internalized ADAM17. Hence, PACS-2 sustains ADAM17 cell-surface activity by diverting ADAM17 away from degradative pathways. Interestingly, Pacs2 -deficient mice display significantly reduced levels of phosphorylated EGFR and intestinal proliferation. We suggest that this mechanism controlling ADAM17 cell-surface availability and EGFR signalling may play a role in intestinal homeostasis, with potential implications for cancer biology. The transmembrane a disintegrin and metalloproteinase 17 (ADAM17, also known as tumour necrosis factor-α (TNF-α)-converting enzyme) promotes intercellular communication by releasing membrane-anchored growth factors, cytokines, receptors and adhesion molecules from cells [1] . Notably, ADAM17 sheds ErbB ligands, enabling activation of ErbB family members on target cells to stimulate epithelial development, growth, regeneration and tumour progression [2] . ADAM17 expression is highly elevated in several human cancers [3] , and inhibition of ADAM17-mediated shedding or genetic ablation of Adam17 reduces tumourigenesis in vivo [4] , [5] . These findings have spurred interest in supplementing clinical Erb1 (also known as epidermal growth factor receptor (EGFR)) inhibition with synergistic targeting of ADAM17 (ref. 1 ). Unfortunately, specific targeting of ADAM17 catalytic activity has proven difficult due to high homology of the ADAM17 active site to other metalloproteinases [1] . Alternatively, interference with the subcellular localization of ADAM17 could provide a novel approach to selectively controlling its activity. A better understanding of ADAM17 regulation is therefore needed. While ADAM17 may act in intracellular compartments, its major shedding activity appears to require localization to the cell surface [6] , [7] , [8] , [9] . Nevertheless, the protease is restricted largely to perinuclear compartments, suggesting that the cell-surface pool of ADAM17 is tightly regulated [10] . Transmembrane cell-surface proteins can be regulated by intracellular trafficking, including internalization from the cell surface and subsequent degradation or recycling back to the cell surface [11] . ADAM17 is regulated by trafficking steps, including control of endoplasmic reticulum (ER) exit by iRhom1/2 (refs. 12 , 13 , 14 ), proteolytic maturation by removal of the ADAM17 prodomain in the trans-Golgi network by furin [10] and stimulation of ADAM17 surface translocation by mitogen-activated protein kinases [15] , [16] . Once at the cell surface, ADAM17 can be activated rapidly through conformational alterations [17] , [18] , [19] . However, ADAM17 maturation is slow, and mature ADAM17 has a long half-life [10] , [20] , suggesting that a mechanism acutely regulating ADAM17 cell-surface availability must exist. Here, we report the results of a functional genome-wide screen identifying phosphofurin acidic cluster sorting protein 2 (PACS-2) as a regulator of ADAM17-mediated shedding. PACS-2 is a multifunctional sorting protein, which interacts with several cargo molecules to mediate, for example, retrograde trafficking from endosomes and from the Golgi [21] , [22] , [23] , [24] , [25] . We demonstrate that PACS-2 controls ADAM17 cell-surface availability, shedding of ErbB ligands and EGFR activity in vivo . Genome-wide screen identifies PACS-2 as an ADAM17 regulator To identify genes that regulate ADAM17-mediated shedding, we screened a whole-genome human siRNA library (see Supplementary Information for an extensive description of the screen). The 21,121 genes covered by the library were individually targeted by pools of 4 siRNAs. Each pool was transfected into quadruplicate wells of HT1080 fibrosarcoma cells stably expressing alkaline phosphatase-tagged pro-heparin-binding EGF-like growth factor (AP-HB-EGF). HT1080 cells express low levels of endogenous HB-EGF and exhibit high knockdown efficiency, making them a suitable model system. Cells were treated with phorbol 12-myristate 13-acetate (PMA), which is a potent ADAM17 activator. In this system, PMA-induced shedding is protein kinase C-α (PKC-α)-dependent, mediated exclusively by ADAM17, and can be measured by loss of AP cell-surface staining [26] ( Fig. 1a ). Stringent selection criteria identified 645 genes, whose knockdown inhibited loss of AP cell-surface staining in response to PMA treatment ( Supplementary Fig. 1a,b ). These genes were then evaluated in a deconvolution screen, where individual siRNAs constituting the original pools were tested separately. By setting a threshold at which at least three of the four individual siRNAs prevented loss of AP surface staining after PMA treatment, 81 genes, including ADAM17 and PKC-α, were validated ( Supplementary Fig. 1c,d and Supplementary Data 1 ). 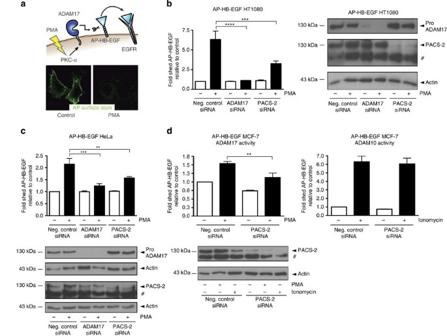Figure 1: Genome-wide screen identifies PACS-2 as an ADAM17 regulator. (a) Cellular model system used for the genome-wide siRNA screen. A total of 21,121 individual genes were knocked down using siRNAs and the effects on ADAM17-mediated shedding of AP-HB-EGF were measured by quantifying AP cell-surface staining after PMA stimulation. (b,c) siRNA-transfected AP-HB-EGF HT1080 (b) or AP-HB-EGF HeLa (c) cells were PMA-stimulated, and the cell medium was analysed for AP activity. The fold change in AP-HB-EGF release was calculated by setting the unstimulated negative control for each experiment to 1, then normalizing the other raw data to this value, and finally calculating the average of all individual experiments. Data inbwere compiled from six individual experiments and incfrom three individual experiments, each performed in triplicate. (d) AP-HB-EGF MCF-7 cells were siRNA-transfected and stimulated with PMA (left-hand panel) or ionomycin (right-hand panel). Conditioned medium was analysed for AP activity as inbandc. Data were compiled from four individual experiments, each performed in triplicate. In all cases, knockdown was confirmed by western blot. On blots, # denotes a nonspecific band. Graphs show mean values±s.e.m. Data were analysed by analysis of variance. **P<0.01, ***P<0.001, ****P<0.0001. Figure 1: Genome-wide screen identifies PACS-2 as an ADAM17 regulator. ( a ) Cellular model system used for the genome-wide siRNA screen. A total of 21,121 individual genes were knocked down using siRNAs and the effects on ADAM17-mediated shedding of AP-HB-EGF were measured by quantifying AP cell-surface staining after PMA stimulation. ( b , c ) siRNA-transfected AP-HB-EGF HT1080 ( b ) or AP-HB-EGF HeLa ( c ) cells were PMA-stimulated, and the cell medium was analysed for AP activity. The fold change in AP-HB-EGF release was calculated by setting the unstimulated negative control for each experiment to 1, then normalizing the other raw data to this value, and finally calculating the average of all individual experiments. Data in b were compiled from six individual experiments and in c from three individual experiments, each performed in triplicate. ( d ) AP-HB-EGF MCF-7 cells were siRNA-transfected and stimulated with PMA (left-hand panel) or ionomycin (right-hand panel). Conditioned medium was analysed for AP activity as in b and c . Data were compiled from four individual experiments, each performed in triplicate. In all cases, knockdown was confirmed by western blot. On blots, # denotes a nonspecific band. Graphs show mean values±s.e.m. Data were analysed by analysis of variance. ** P <0.01, *** P <0.001, **** P <0.0001. Full size image Computational algorithms segregated the screen hits into multiple categories and no enrichment in particular signalling pathways was evident ( Supplementary Fig. 1e ; Supplementary Data 1 ). Hits were further evaluated using an independent shedding assay, where release of AP-HB-EGF into the cell medium was quantified by addition of a colorimetric AP substrate. This revealed that knockdown of 24 genes mimicked the effects of ADAM17 knockdown on AP-HB-EGF shedding ( Supplementary Data 1 ). Among these were the multifunctional sorting protein PACS-2 (Library gene ID KIAA0602; GenBank BC050351). In AP-HB-EGF HT1080 cells, knockdown of PACS-2 significantly inhibited PMA-stimulated shedding mediated by ADAM17 ( Fig. 1b ). Owing to the apparent importance of trafficking for the ADAM17 life cycle, we selected PACS-2 for further analysis. PACS-2 regulates ADAM17-mediated shedding As PACS-2 knockdown showed an inhibitory effect on ADAM17-mediated shedding in the functional genome-wide screen, we next validated the effect of PACS-2 knockdown in other contexts. Firstly, we observed the same inhibitory effect of PACS-2 knockdown on shedding in AP-HB-EGF HT1080 cells using an independent set of siRNAs from another manufacturer ( Supplementary Fig. 2a ). PACS-2 siRNA did not knock down the structurally related PACS-1 ( Supplementary Fig. 2b ). Validating our finding from the screen in two other cell lines, PACS-2 knockdown also inhibited PMA-stimulated shedding mediated by ADAM17 in AP-HB-EGF-expressing HeLa and MCF-7 cells ( Fig. 1c,d ). Importantly, knockdown of PACS-2 affected neither the cell-surface levels of AP-HB-EGF in HT1080 cells ( Supplementary Fig. 3a ) nor the total cellular expression of AP-HB-EGF in any of the cell lines used ( Supplementary Fig. 3b–d ), indicating that the inhibitory effects of PACS-2 knockdown on ADAM17-mediated shedding were not caused by decreased substrate availability. While PMA treatment induces ADAM17-mediated shedding in AP-HB-EGF MCF-7 cells, stimulation of this cell line with the calcium ionophore ionomycin has been shown to selectively activate ADAM10ref. [27] , the closest ADAM17 relative. This cell line thereby allows us to distinguish effects on ADAM17 from effects on ADAM10. By stimulating AP-HB-EGF MCF-7 cells with ionomycin, we showed that PACS-2 knockdown had no effect on ADAM10-mediated shedding ( Fig. 1d ). This indicates that PACS-2 regulates ADAM17 with some selectivity. For unknown reasons, treatment with ionomycin led to a reduction of PACS-2 levels. As ADAM17 is also the prominent PMA-responsive sheddase in mouse embryonic fibroblasts (MEFs) [28] , we examined the effects of Pacs2 -deficiency on PMA-induced shedding of AP-HB-EGF in control and Pacs2 −/− MEFs [24] . We found that Pacs2 −/− MEFs exhibited significantly lower shedding in response to PMA treatment than control MEFs ( Fig. 2a ). The decreased shedding from Pacs2 −/− MEFs was rescued by re-expression of exogenous PACS-2, confirming the importance of PACS-2 for ADAM17-mediated shedding ( Fig. 2b ). 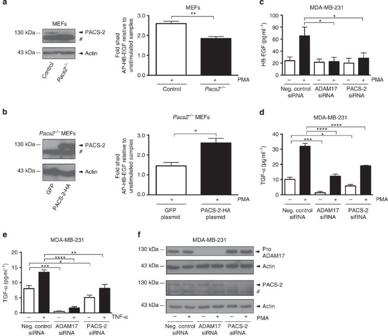Figure 2: PACS-2 regulates ADAM17-mediated shedding. (a) AP-HB-EGF was transiently expressed in control andPacs2−/−MEFs. Cells were PMA-stimulated, and the cell medium was analysed for AP activity. To overcome differences in transfection efficiency, the fraction of shed AP-HB-EGF was calculated as AP-HB-EGF released to the medium divided by the total amount of AP-HB-EGF in the medium and cell lysate. The fold change in AP-HB-EGF release was then calculated by setting the unstimulated negative control for each experiment to 1, normalizing the other raw data to this value and finally calculating the average of all individual experiments. The PMA-stimulated fold increase in AP-HB-EGF shedding was depicted for each cell line. Data were compiled from four individual experiments, each performed in triplicate. (b) AP-HB-EGF was expressed inPacs2−/−MEFs together with green fluorescent protein (GFP) or PACS-2-HA and shedding analysed as ina. Data were compiled from three individual experiments, each performed in triplicate. (c–e) siRNA-transfected MDA-MB-231 cells were stimulated with PMA (c,d) or TNF-α (e). The medium was analysed by ELISA for shed HB-EGF (c) or TGF-α (d,e), shown as concentrations in pg ml−1. In all cases, data were compiled from three individual experiments, each performed in triplicate. (f) Representative western blots showing knockdown in cells used for ELISA. On blots, # denotes a nonspecific band. Graphs show mean values±s.e.m. Data were analysed by analysis of variance or unpaired two-tailed Student’st-test, as appropriate. *P<0.05, **P<0.01, ***P<0.001, ****P<0.0001. Figure 2: PACS-2 regulates ADAM17-mediated shedding. ( a ) AP-HB-EGF was transiently expressed in control and Pacs2 −/− MEFs. Cells were PMA-stimulated, and the cell medium was analysed for AP activity. To overcome differences in transfection efficiency, the fraction of shed AP-HB-EGF was calculated as AP-HB-EGF released to the medium divided by the total amount of AP-HB-EGF in the medium and cell lysate. The fold change in AP-HB-EGF release was then calculated by setting the unstimulated negative control for each experiment to 1, normalizing the other raw data to this value and finally calculating the average of all individual experiments. The PMA-stimulated fold increase in AP-HB-EGF shedding was depicted for each cell line. Data were compiled from four individual experiments, each performed in triplicate. ( b ) AP-HB-EGF was expressed in Pacs2 −/− MEFs together with green fluorescent protein (GFP) or PACS-2-HA and shedding analysed as in a . Data were compiled from three individual experiments, each performed in triplicate. ( c – e ) siRNA-transfected MDA-MB-231 cells were stimulated with PMA ( c , d ) or TNF-α ( e ). The medium was analysed by ELISA for shed HB-EGF ( c ) or TGF-α ( d , e ), shown as concentrations in pg ml −1 . In all cases, data were compiled from three individual experiments, each performed in triplicate. ( f ) Representative western blots showing knockdown in cells used for ELISA. On blots, # denotes a nonspecific band. Graphs show mean values±s.e.m. Data were analysed by analysis of variance or unpaired two-tailed Student’s t -test, as appropriate. * P <0.05, ** P <0.01, *** P <0.001, **** P <0.0001. Full size image To evaluate the functional interaction between PACS-2 and ADAM17 using endogenously expressed ADAM17 substrates, we performed PACS-2 knockdown in MDA-MB-231 breast carcinoma cells, which express detectable levels of HB-EGF and transforming growth factor-α (TGF-α). Cells were left unstimulated or treated with PMA, and the conditioned medium assayed for shed HB-EGF and TGF-α using enzyme-linked immunosorbent assays (ELISAs). In agreement with the alkaline phosphatase reporter assays, PACS-2 knockdown mimicked ADAM17 loss also with regard to endogenous substrates. In MDA-MB-231 cells, PMA-stimulated HB-EGF shedding was highly ADAM17-dependent, whereas unstimulated HB-EGF shedding was not mediated by ADAM17. Accordingly, PACS-2 knockdown significantly reduced PMA-stimulated shedding of endogenous HB-EGF without affecting basal shedding ( Fig. 2c ). ADAM17 was required for basal TGF-α shedding, and partially for PMA-stimulated TGF-α shedding. Again, PACS-2 knockdown mimicked the effects of ADAM17 knockdown by statistically significantly reducing both basal and stimulated shedding ( Fig. 2d ). This was also the case when evaluating TGF-α shedding induced by the physiological stimulant TNF-α ( Fig. 2e ). Knockdown was confirmed by western blot on cells used for ELISA ( Fig. 2f ). Thus, PACS-2 regulates ADAM17-mediated shedding of different substrates in numerous cell types under unstimulated, as well as stimulated conditions. PACS-2 regulates cell-surface availability of mature ADAM17 Since PACS-2 regulated ADAM17-mediated shedding under basal as well as stimulated conditions, we speculated that PACS-2 could be controlling ADAM17 levels, and thereby sheddase activity. The ADAM17 proenzyme is synthesized in the ER, and during transit to the cell surface, furin-mediated cleavage in the trans-Golgi network generates the mature and enzymatically active ADAM17 (refs. 10 , 29 ). To investigate to what extent PACS-2 knockdown affects ADAM17 levels and cell-surface exposure, we performed cell-surface biotinylation on MDA-MB-231 cells. Interestingly, PACS-2 knockdown caused a statistically significant decrease in the level of cell-surface biotinylated ADAM17 ( Fig. 3a ). Western blot analysis of total cell lysates further revealed that PACS-2 knockdown reduced the total level of mature ADAM17 without significantly affecting the proenzyme ( Fig. 3b ). As previously reported, high-dose PMA treatment results in a rapid activation of ADAM17, followed by subsequent downregulation of ADAM17 by endocytosis [20] . This effect was seen here by decreased ADAM17 levels both on the cell surface ( Fig. 3a ) and in total cell lysates ( Fig. 3b ) after PMA stimulation, and was also evident in PACS-2-deficient cells where mature ADAM17 levels are low independently of PMA treatment. 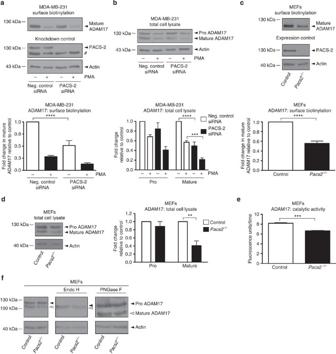Figure 3: PACS-2 regulates cell-surface availability of mature ADAM17. (a,b) MDA-MB-231 cells were siRNA-transfected and PMA-stimulated. Cells were surface biotinylated and analysed by western blot. ADAM17 levels were normalized to input actin and fold changes were calculated by setting the unstimulated negative control for each experiment to 1, then normalizing the other raw data to this value and finally calculating the average of all individual experiments. Cell-surface levels of mature ADAM17 (a) and total cellular levels of pro and mature ADAM17 (b) are shown with data compiled from four individual experiments. (c,d) Unstimulated cell-surface levels of mature ADAM17 (c) and total cellular levels of pro and mature ADAM17 (d) in control andPacs2−/−MEFs were analysed as inaandb. Data were compiled from four individual experiments incand three individual experiments ind. (e) ADAM17 was immunoprecipitated from unstimulated control andPacs2−/−MEFs and its activity assessed using an ADAM17 quenched fluorescence peptide substrate. The graph shows the average gradient (fluorescence units/time) of the linear regressions describing enzymatic activity. The data were compiled from three individual experiments, each performed in triplicate. (f) Lysates from control andPacs2−/−MEFs were treated with EndoH or PNGase F and the effects on ADAM17 examined by western blot. The images shown are derived from the same blot but different exposures (indicated by separate panels). The blot shown is representative of three individual experiments. On blots, # denotes a nonspecific band. Graphs show mean values±s.e.m. Data were analysed by analysis of variance or unpaired two-tailed Student’st-test, as appropriate. **P<0.01, ***P<0.001, ****P<0.0001. Figure 3: PACS-2 regulates cell-surface availability of mature ADAM17. ( a , b ) MDA-MB-231 cells were siRNA-transfected and PMA-stimulated. Cells were surface biotinylated and analysed by western blot. ADAM17 levels were normalized to input actin and fold changes were calculated by setting the unstimulated negative control for each experiment to 1, then normalizing the other raw data to this value and finally calculating the average of all individual experiments. Cell-surface levels of mature ADAM17 ( a ) and total cellular levels of pro and mature ADAM17 ( b ) are shown with data compiled from four individual experiments. ( c , d ) Unstimulated cell-surface levels of mature ADAM17 ( c ) and total cellular levels of pro and mature ADAM17 ( d ) in control and Pacs2 −/− MEFs were analysed as in a and b . Data were compiled from four individual experiments in c and three individual experiments in d . ( e ) ADAM17 was immunoprecipitated from unstimulated control and Pacs2 −/− MEFs and its activity assessed using an ADAM17 quenched fluorescence peptide substrate. The graph shows the average gradient (fluorescence units/time) of the linear regressions describing enzymatic activity. The data were compiled from three individual experiments, each performed in triplicate. ( f ) Lysates from control and Pacs2 −/− MEFs were treated with EndoH or PNGase F and the effects on ADAM17 examined by western blot. The images shown are derived from the same blot but different exposures (indicated by separate panels). The blot shown is representative of three individual experiments. On blots, # denotes a nonspecific band. Graphs show mean values±s.e.m. Data were analysed by analysis of variance or unpaired two-tailed Student’s t -test, as appropriate. ** P <0.01, *** P <0.001, **** P <0.0001. Full size image To validate these findings obtained using siRNA against PACS-2, we performed similar experiments on control and Pacs2 -deficient MEFs and found that Pacs2 −/− MEFs likewise had significantly reduced amounts of mature ADAM17 on the cell surface, as well as in total cell lysates, where there was again no significant effect on the ADAM17 proform ( Fig. 3c,d ). To assay ADAM17 catalytic activity, ADAM17 from control and Pacs2 −/− MEFs was first captured and then incubated with a quenched fluorescence peptide substrate. This revealed that the observed decrease in mature ADAM17 levels in Pacs2 −/− MEFs was indeed reflected in a lower rate of catalytic activity ( Fig. 3e ). Importantly, PACS-2 knockdown had no statistically significant effects on cell-surface levels of the related metalloproteinases ADAM9, membrane-type 1 matrix metalloproteinase (MT1-MMP), ADAM10, or on the EGFR, further supporting the notion that PACS-2 selectively regulates ADAM17 ( Supplementary Fig. 4 , and see Fig. 1d ). PACS-2 mediates trafficking between multiple cellular compartments [21] , [22] , [23] , [24] , [25] , and could therefore regulate ADAM17 in several ways. As one possibility, the observed decrease in mature ADAM17 levels could result from disrupted ADAM17 maturation. To test this, we treated lysates from control and Pacs2 −/− MEFs with Endoglycosidase H (EndoH) or Peptide-N-glycosidase F (PNGase F). N-linked glycosylations added in the ER become EndoH resistant after being modified in the Golgi apparatus. In contrast, PNGase treatment removes all N-linked glycosylations. As it has previously been shown [10] , ER-resident ADAM17 proform from control cells was EndoH sensitive whereas the surface-localized mature form was resistant. As expected, PNGase treatment led to a reduction in size of both forms. Importantly, ADAM17 from Pacs2 −/− MEFs showed the same sensitivity to EndoH and PNGase treatment as ADAM17 from control MEFs, although in total, less mature ADAM17 was present ( Fig. 3f ). This indicates that Pacs2 -deficiency does not cause ER retention of ADAM17. PACS-2 interacts with ADAM17 in endocytic compartments To further investigate how PACS-2 regulates ADAM17 cell-surface levels, we asked whether the two proteins interact. Co-immunoprecipitation experiments revealed an interaction of PACS-2 with the mature form of ADAM17 in both unstimulated and PMA-stimulated cells ( Fig. 4a,b ). We confirmed the identity of the co-immunoprecipitated PACS-2 band by repeating the experiment in MEFs, where no co-immunoprecipitation was seen in Pacs2 −/− cells ( Supplementary Fig. 5 ). Quantification of the co-immunoprecipitated bands showed no significant differences in intensities between unstimulated and PMA-stimulated cells in either MDA-MB-231 or control MEFs ( Fig. 4c and Supplementary Fig. 5b ). 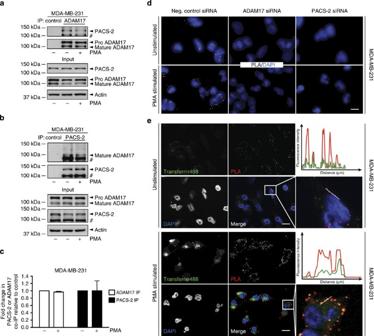Figure 4: PACS-2 interacts with ADAM17 in endocytic compartments. (a,b) ADAM17 (a) or PACS-2 (b) was immunoprecipitated (IP) from unstimulated and PMA-stimulated MDA-MB-231 cells, and co-immunoprecipitation (co-IP) of PACS-2 (a) or ADAM17 (b) detected by western blot. The blots shown are representative of three individual experiments and # denotes a nonspecific band. (c) The effect of PMA stimulation on PACS-2/ADAM17 co-immunoprecipitation inaandbwas quantified. The amount of co-immunoprecipitated PACS-2 (a) or mature ADAM17 (b) was normalized to the amount of immunoprecipitated mature ADAM17 (a) or PACS-2 (b). The unstimulated negative control for each experiment was then set to 1, the other raw data were normalized to this value and finally the average of all individual experiments was calculated. Data were analysed by unpaired two-tailed Student’st-test. (d) MDA-MB-231 cells were transfected with siRNA and subjected to PLA with or without PMA stimulation. The experiment was performed 10 times in duplicate. Two experiments included the knockdown controls. Scale bar, 7 μm. (e) Before PLA, MDA-MB-231 cells were left unstimulated or treated with PMA and subsequently allowed to internalize fluorescent transferrin for 5 min. Scale bar, 14 μm. Fluorescence intensities were quantified along the lines on the enlarged images and depicted on the graphs. The experiment was performed four times in duplicate. Figure 4: PACS-2 interacts with ADAM17 in endocytic compartments. ( a , b ) ADAM17 ( a ) or PACS-2 ( b ) was immunoprecipitated (IP) from unstimulated and PMA-stimulated MDA-MB-231 cells, and co-immunoprecipitation (co-IP) of PACS-2 ( a ) or ADAM17 ( b ) detected by western blot. The blots shown are representative of three individual experiments and # denotes a nonspecific band. ( c ) The effect of PMA stimulation on PACS-2/ADAM17 co-immunoprecipitation in a and b was quantified. The amount of co-immunoprecipitated PACS-2 ( a ) or mature ADAM17 ( b ) was normalized to the amount of immunoprecipitated mature ADAM17 ( a ) or PACS-2 ( b ). The unstimulated negative control for each experiment was then set to 1, the other raw data were normalized to this value and finally the average of all individual experiments was calculated. Data were analysed by unpaired two-tailed Student’s t -test. ( d ) MDA-MB-231 cells were transfected with siRNA and subjected to PLA with or without PMA stimulation. The experiment was performed 10 times in duplicate. Two experiments included the knockdown controls. Scale bar, 7 μm. ( e ) Before PLA, MDA-MB-231 cells were left unstimulated or treated with PMA and subsequently allowed to internalize fluorescent transferrin for 5 min. Scale bar, 14 μm. Fluorescence intensities were quantified along the lines on the enlarged images and depicted on the graphs. The experiment was performed four times in duplicate. Full size image To further study the PACS-2/ADAM17 interaction, we turned to Proximity Ligation Assay (PLA), a highly sensitive technique for the detection of closely co-localized proteins. This method has the advantage that it reveals protein–protein interactions in situ , without the substantial manipulations involved in immunoprecipitation [30] . PLA showed co-localization of endogenous ADAM17 and PACS-2 in unstimulated MDA-MB-231 cells ( Fig. 4d ). The PLA co-localization signal was abolished by knockdown of either PACS-2 or ADAM17, indicating its specificity. Interestingly, PMA treatment increased the PLA signal ( Fig. 4d ), suggesting an enhanced PACS-2/ADAM17 interaction that is lost during co-immunoprecipitation. As described, high-dose PMA treatment, used here and in the previous figures, enhances ADAM17 internalization ( [20] and see Fig. 3a,b ). We therefore tested whether a lower dose of PMA had a similar effect. PACS-2 knockdown also decreased shedding induced by low-dose PMA treatment ( Supplementary Fig. 6a ), but this dose was less effective at enhancing PACS-2/ADAM17 co-localization ( Supplementary Fig. 6b ). Thus, this dose-dependent enhancement of the PLA signal suggested that the interaction occurs upon ADAM17 endocytosis. Indeed, the PACS-2/ADAM17 co-localization by PLA overlapped with internalized fluorescent transferrin in early endosomes, in unstimulated, as well as PMA-stimulated cells ( Fig. 4e ). Together with the immunoprecipitation studies showing interaction of PACS-2 with mature ADAM17, these findings suggest that PACS-2 interacts with ADAM17 in early endocytic compartments. The interaction occurs irrespective of PMA treatment; yet, as revealed using the highly sensitive PLA method, the PACS-2/ADAM17 interaction may be further induced by stimulating ADAM17 endocytosis with high-dose PMA. PACS-2 diverts ADAM17 away from degradative pathways On the basis of the observed co-localization of PACS-2 and ADAM17 on early endosomes, we asked whether PACS-2 affects ADAM17 endocytosis. By labelling cell-surface proteins with cleavable biotin and allowing these to be internalized and recycled, we found that although PACS-2 knockdown reduced basal ADAM17 cell-surface levels, it did not alter the efficiency of constitutive ADAM17 internalization (calculated relative to initial total cell-surface levels). However, PACS-2 knockdown caused a small but statistically significant decrease in ADAM17 recycling during the time measured (calculated as a percentage of internalized protein, Fig. 5a ). We furthermore assessed protein stability by cell-surface labelling MDA-MB-231 cells with non-cleavable biotin and tracing the amount of biotinylated protein remaining after 4 h of incubation. Here, PACS-2 knockdown resulted in increased loss of biotinylated ADAM17 ( Fig. 5b ). Together, these findings suggest that PACS-2 controls the cell-surface availability of ADAM17 by diverting the endocytosed sheddase away from degradative pathways. 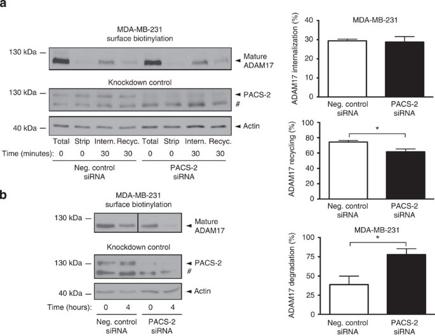Figure 5: PACS-2 diverts endocytosed ADAM17 away from degradative pathways. (a) MDA-MB-231 cells were surface labelled using cleavable biotin. Labelled cell-surface proteins were allowed to internalize for 30 min and remaining biotinylated proteins on the cell surface were removed (Intern.). Internalized proteins were then allowed to recycle for 30 min, after which recycled protein was stripped from the cell surface (Recyc.). The amount of cell-surface ADAM17 was first normalized to input actin. The percentage internalization was calculated relative to total cell-surface ADAM17 levels (Total). Recycling was determined by first subtracting the amount of biotinylated protein left after recycling from the amount of internalized protein, and then calculated as a percentage of internalized protein. To verify proper stripping of cell-surface proteins, a dish kept at 4 °C was processed in parallel (Strip). Data were compiled from five individual experiments. (b) MDA-MB-231 cells were surface labelled using non-cleavable biotin, lysed at time zero, or incubated for 4 h at 37 °C to allow internalization and degradation of surface proteins. Percentage degradation was calculated by normalizing the amount of cell-surface ADAM17 to input actin, and dividing the amount remaining after 4 h with the amount present at time zero. Data were compiled from three individual experiments. The images shown are derived from the same blot and same exposure, but have been cropped for clarity (indicated by a separation line). On blots, # denotes a nonspecific band. Graphs show mean values±s.e.m. Data were analysed by unpaired two-tailed Student’st-test. *P<0.05. Figure 5: PACS-2 diverts endocytosed ADAM17 away from degradative pathways. ( a ) MDA-MB-231 cells were surface labelled using cleavable biotin. Labelled cell-surface proteins were allowed to internalize for 30 min and remaining biotinylated proteins on the cell surface were removed (Intern.). Internalized proteins were then allowed to recycle for 30 min, after which recycled protein was stripped from the cell surface (Recyc.). The amount of cell-surface ADAM17 was first normalized to input actin. The percentage internalization was calculated relative to total cell-surface ADAM17 levels (Total). Recycling was determined by first subtracting the amount of biotinylated protein left after recycling from the amount of internalized protein, and then calculated as a percentage of internalized protein. To verify proper stripping of cell-surface proteins, a dish kept at 4 °C was processed in parallel (Strip). Data were compiled from five individual experiments. ( b ) MDA-MB-231 cells were surface labelled using non-cleavable biotin, lysed at time zero, or incubated for 4 h at 37 °C to allow internalization and degradation of surface proteins. Percentage degradation was calculated by normalizing the amount of cell-surface ADAM17 to input actin, and dividing the amount remaining after 4 h with the amount present at time zero. Data were compiled from three individual experiments. The images shown are derived from the same blot and same exposure, but have been cropped for clarity (indicated by a separation line). On blots, # denotes a nonspecific band. Graphs show mean values±s.e.m. Data were analysed by unpaired two-tailed Student’s t -test. * P <0.05. Full size image PACS-2 controls EGFR activity in vivo Given the effects of PACS-2 on mature ADAM17 levels and shedding of ErbB ligands, we asked how genetic deletion of Pacs2 affects downstream EGFR activation in vivo . Pacs2 −/− mice show no signs of early postnatal lethality, wavy coat, open eyes at birth, or any obvious defects in the skin, which are characteristics of the complete and conditional ADAM17 and EGFR knockouts [31] , [32] , [33] , [34] , [35] , [36] , [37] . However, since EGFR signalling is highly mitogenic for intestinal stem cells [38] , we chose to investigate the Pacs2 −/− intestine. Using an antibody rigorously validated on EGFR knockout mouse tissue [38] , we performed immunohistochemistry for activated EGFR (phosphorylated on Tyr1068, henceforth referred to as pEGFR) on histological sections of the small intestine from control and Pacs2 -deficient mice. Interestingly, we found that levels of pEGFR in small intestinal crypts were significantly reduced in Pacs2 −/− mice ( Fig. 6a,b ). Supporting this observation, western blot on crude small intestinal lysates from control and Pacs2 −/− mice showed significantly reduced pEGFR levels, while no change in total EGFR expression was found ( Supplementary Fig. 7a ). To uncover potential cell-autonomous effects on EGFR activation, control and Pacs2 −/− MEFs were deprived of exogenous growth factors by serum starvation. As shown by western blot analysis, there was no difference in total EGFR expression, but the level of pEGFR was significantly reduced in Pacs2 -deficient cells as compared with wild-type control ( Supplementary Fig. 7b ). Together, these findings indicate that PACS-2 regulates EGFR activity in vivo . 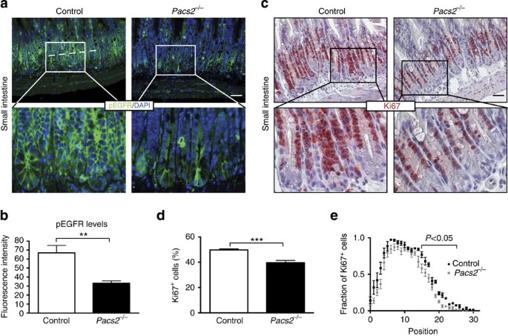Figure 6: PACS-2 controls EGFR activityin vivo. (a) Immunohistochemistry for EGFR pY1068 and nuclear DAPI stain were performed on sections from the small intestine of five wild-type and sevenPacs2−/−mice. Scale bar, 43 μm. (b) For each section, four images were taken at corresponding random points and the fluorescence intensity of pEGFR quantified along a line averaging 193 μm across small intestinal crypts, represented by the dotted line ina. (c) Immunohistochemistry for Ki67 on sections from the small intestine of five control and sixPacs2−/−mice. Scale bar, 52 μm. (d) The percentage of Ki67-positive cells was quantified. For each mouse, over 900 crypt cells were scored, unless not enough well-oriented crypts were available. (e) The position of Ki67-positive cells in small intestinal crypts was scored from crypt-cell position 0 (bottom) to 30 (top) and the number represented as a fraction out of the total number of cells counted for each position. Graphs show mean values±s.e.m. Data were analysed by unpaired two-tailed Student’st-test. **P<0.01, ***P<0.001. Figure 6: PACS-2 controls EGFR activity in vivo . ( a ) Immunohistochemistry for EGFR pY1068 and nuclear DAPI stain were performed on sections from the small intestine of five wild-type and seven Pacs2 −/− mice. Scale bar, 43 μm. ( b ) For each section, four images were taken at corresponding random points and the fluorescence intensity of pEGFR quantified along a line averaging 193 μm across small intestinal crypts, represented by the dotted line in a . ( c ) Immunohistochemistry for Ki67 on sections from the small intestine of five control and six Pacs2 −/− mice. Scale bar, 52 μm. ( d ) The percentage of Ki67-positive cells was quantified. For each mouse, over 900 crypt cells were scored, unless not enough well-oriented crypts were available. ( e ) The position of Ki67-positive cells in small intestinal crypts was scored from crypt-cell position 0 (bottom) to 30 (top) and the number represented as a fraction out of the total number of cells counted for each position. Graphs show mean values±s.e.m. Data were analysed by unpaired two-tailed Student’s t -test. ** P <0.01, *** P <0.001. Full size image PACS-2 regulates intestinal homeostasis Signalling via the EGFR pathway is linked to intestinal cell proliferation and tissue homeostasis [38] . Importantly, the reduced pEGFR levels found in the small intestine of Pacs2 −/− mice were coupled with a statistically significant decrease in the number of proliferating crypt cells, determined by Ki67 staining ( Fig. 6c,d ). An assessment of the relative positions of Ki67-positive cells revealed that this decrease primarily affected the higher crypt-cell positions, resulting in a shorter proliferative zone of small intestinal crypts in Pacs2 −/− mice ( Fig. 6e ). An investigation of colon sections from Pacs2 −/− mice showed similarly decreased levels of pEGFR ( Supplementary Fig. 8a,b ), and a tendency towards a decreased number of Ki67-positive cells ( Supplementary Fig. 8c–e ). In addition to the reduced cell proliferation, the small intestine of Pacs2 −/− mice displayed a decreased villus to crypt ratio compared with control mice ( Fig. 7a,b ). No significant difference in crypt depth was observed in the colon of Pacs2 -deficient mice ( Supplementary Fig. 8f,g ). These findings suggest that PACS-2 regulates EGFR activity and may contribute to intestinal homeostasis. 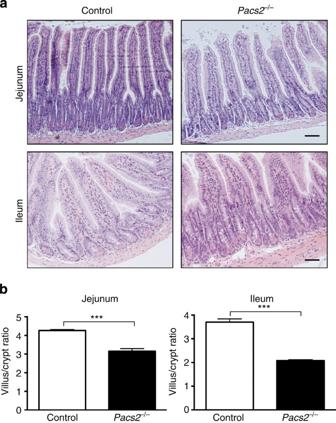Figure 7: PACS-2 regulates intestinal tissue homeostasis. (a) Histology of the small intestine ofPacs2−/−mice. Scale bars, 63 μm. (b) The ratio of villus height to crypt depth in jejunum and ileum was quantified using four control and fourPacs2−/−mice. More than 100 villi were assessed for each genotype and segment. Graphs show mean values±s.e.m. Data were analysed by unpaired two-tailed Student’st-test. ***P<0.001. Figure 7: PACS-2 regulates intestinal tissue homeostasis. ( a ) Histology of the small intestine of Pacs2 −/− mice. Scale bars, 63 μm. ( b ) The ratio of villus height to crypt depth in jejunum and ileum was quantified using four control and four Pacs2 −/− mice. More than 100 villi were assessed for each genotype and segment. Graphs show mean values±s.e.m. Data were analysed by unpaired two-tailed Student’s t -test. *** P <0.001. Full size image ADAM17-mediated shedding of ErbB ligands is critical for intracellular signalling controlling development, growth and tumour progression. Here, we identify PACS-2-mediated control of ADAM17 cell-surface availability as an important regulator of ADAM17 and EGFR activity. By interacting with ADAM17 in endocytic compartments and diverting endocytosed ADAM17 away from degradative pathways, PACS-2 acts to maintain mature ADAM17 levels and sustain sheddase activity. We propose that in this way, PACS-2 regulates the strength of ErbB signalling ( Fig. 8 ). 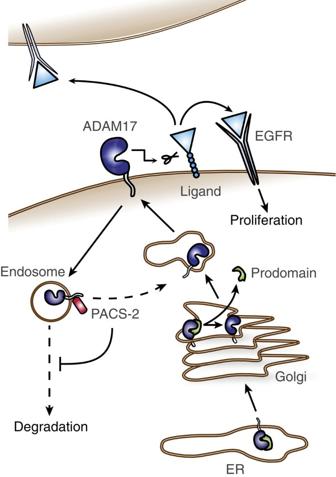Figure 8: A model of PACS-2 regulation of ADAM17 and EGFR activity. The ADAM17 proform mainly resides in the secretory apparatus, and during its transit to the cell surface, furin-mediated cleavage generates the mature (active) form. We propose that PACS-2 controls ADAM17 cell-surface availability by diverting endocytosed ADAM17 away from degradative pathways and towards sustained ErbB ligand shedding and EGFR activation. PACS-2 is therefore an important regulator of auto, para and juxtacrine ErbB signallingin vivo. Figure 8: A model of PACS-2 regulation of ADAM17 and EGFR activity. The ADAM17 proform mainly resides in the secretory apparatus, and during its transit to the cell surface, furin-mediated cleavage generates the mature (active) form. We propose that PACS-2 controls ADAM17 cell-surface availability by diverting endocytosed ADAM17 away from degradative pathways and towards sustained ErbB ligand shedding and EGFR activation. PACS-2 is therefore an important regulator of auto, para and juxtacrine ErbB signalling in vivo . Full size image PACS-2 sorts a number of cargo molecules between intracellular compartments [21] , [22] , [23] , [24] , [25] . For example, PACS-2 has been previously detected in endosomes mediating retrograde cargo trafficking [21] . Similarly, we found that PACS-2 interacted with mature ADAM17, and that PACS-2/ADAM17 co-localization overlapped substantially with transferrin-positive early endosomes. PACS-2 loss did not affect constitutive ADAM17 internalization, but rather decreased the cell-surface recycling and stability of internalized ADAM17. While the effect of PACS-2 on ADAM17 recycling may seem relatively small, the magnitude is comparable to what has been reported for other endocytic regulators [39] . Although PACS-2 appears to control the endocytic fate of ADAM17, PACS-2 and ADAM17 are both found in the ER [10] , [40] and may interact there too. Yet, Pacs2 -deficient MEFs showed similar sensitivity of ADAM17 to deglycosylation enzymes as did control MEFs. Moreover, in both MEF and MDA-MB-231 cells, loss of PACS-2 caused a significant reduction in the mature form of ADAM17 without affecting the amount of proform. Together, this suggests that loss of PACS-2 does not lead to ADAM17 retention in the ER or altered protein secretion. The phorbol ester PMA is a well-known activator of ADAM17, acting through mitogen-activated protein kinase and/or PKC pathways [26] , [41] . In the present study, we used PMA treatment to selectively induce ADAM17-mediated shedding of ErbB ligands. While loss of PACS-2 reduces PMA-stimulated ADAM17-mediated shedding of several substrates, we have no indications that PACS-2 regulation of ADAM17 is PMA-dependent. On the contrary, loss of PACS-2 results in reduced levels of mature ADAM17 on the cell surface of unstimulated cells, and interaction of PACS-2 with ADAM17 is also seen under these basal conditions. The observed reduction in PMA-induced shedding is therefore likely a result of less mature protease being available for activation. Supporting this, using a quenched fluorescence peptide activity assay, we observed a decrease in basal ADAM17 catalytic activity in Pacs2 -deficient MEFs. PACS-2 frequently binds an acidic cluster motif in its cargo molecules [25] . Although no acidic cluster is found in the cytoplasmic tail of ADAM17, both co-immunoprecipitation and PLA experiments clearly show that PACS-2 interacts with ADAM17 under basal conditions. While PACS-2 can also bind cargo through other motifs [22] , this could suggest that PACS-2 may not bind directly to ADAM17. Our PLA data indicate that the PACS-2/ADAM17 interaction is enhanced upon treatment with PMA, which apart from enhancing ADAM17 internalization also activates intracellular signalling. This finding raises the question whether the interaction is somehow regulated in response to signalling pathways activated by PMA treatment. It is known that Akt kinase can phosphorylate PACS-2, shifting it from a cargo receptor to an apoptotic regulator in response to TRAIL signalling [24] . However, whether PACS-2 is phosphorylated in response to PMA treatment and if this affects its subcellular localization and/or cargo binding awaits further studies. Several PACS-2 transmembrane cargo proteins have been reported [21] , [23] , [42] , [43] , and the regulatory mechanisms of action and compartmental sorting involved vary depending on the cargo molecule. Thus, while PACS-2 does not restrict its activities to ADAM17, our data demonstrate that a number of homologous proteases and the EGFR itself are not similarly affected. How this specificity is conveyed is at present unknown. A potential explanation could simply be that PACS-2 does not interact with ADAM9, MT1-MMP, ADAM10 or EGFR. Furthermore, differences in the intracellular trafficking itinerary of ADAM17 versus the other proteins examined may confer specificity. One could imagine that the route, dynamics, or regulatory machinery of ADAM17 internalization and/or subsequent endosomal fate differ from those of ADAM9, MT1-MMP, ADAM10 and EGFR. PACS-2 could also be directly regulating the substrates of ADAM17 and in this way impact shedding. While dual regulation of both protease and substrate seems to be the case for the ADAM17 regulator iRhom2 (refs 12 , 13 , 44 ), we have no indications that this is the case for PACS-2. In our primary screen, we specifically selected hits with no effect on unstimulated AP-HB-EGF surface levels, and subsequently confirmed that PACS-2 knockdown did not change AP-HB-EGF expression in the cell lines used. Accordingly, PACS-2 knockdown only decreased shedding of AP-tagged as well as endogenous substrates where this is an ADAM17-mediated process. Pacs2 −/− mice exhibit decreased levels of phosphorylated EGFR in the small intestine and colon, supporting a key role for PACS-2 in the regulation of ErbB signalling in vivo . A complete analysis of the Pacs2 −/− mice, both in terms of age and with respect to different tissues has yet to be performed. However, the phenotype of Pacs2 -deficient mice is mild compared with the multi-organ defects observed in Adam17 and Egfr -deficient mice [31] , [32] , [33] , [34] , [35] , [36] , [37] . In contrast to these models, Pacs2 −/− mice still exhibit substantial ADAM17 and EGFR activities, and rather appear to lack a regulatory mechanism to sustain acute ADAM17 activation. Also, PACS-2-mediated regulation of ADAM17 may be more important in some tissues than others, leading to a partial phenotype. We observed that Pacs2 −/− mice have decreased villus/crypt ratio in the small intestine. Interestingly, intestinal abnormalities are seen in a selection of clinical and genetic studies of loss-of-function mutations in the ADAM17/EGFR axis. Specifically, altered intestinal homeostasis was observed in Adam17 knockout mice [31] , triple-null mice lacking EGF, amphiregulin and TGF-α [45] , and in children with a loss-of-function mutation in ADAM17 (ref. 46 ). Furthermore, on a certain genetic background, Egfr −/− mice have similar developmental defects [35] . Although the reported phenotypes are not directly comparable, the similarities are interesting and support the role of PACS-2 as a regulator of ADAM17 and EGFR signalling in vivo . Another model comparable to the Pacs2 −/− mouse is the hypomorphic Adam17 ex/ex mouse, which expresses globally low levels of ADAM17. While the overall phenotype of Adam17 ex/ex mice is more severe than that of the Pacs2 −/− mice, they exhibit no apparent intestinal phenotype [34] . A potential explanation for this discrepancy could be that although the Pacs2 −/− mice express higher ADAM17 levels than Adam17 ex/ex mice, they lack a regulatory mechanism whereby a fraction of already matured ADAM17 can be acutely activated. Possibly, the need for prompt ADAM17-mediated EGFR activation is central in tissues of high turnover, such as the intestinal epithelium. Supporting that ADAM17 levels are not necessarily directly correlated with ADAM17 activity, transgenic mice, which globally overexpress ADAM17, do not show increased ADAM17-shedding activity and have no overt abnormalities [47] . As mentioned above, the intestinal effects of Egfr deletion are highly dependent on genetic background, and several mouse models of EGFR deficiency show no intestinal abnormalities [32] , [33] , [48] . For example, inducible enterocyte-specific deletion of Egfr in adult mice did not affect intestinal tissue homeostasis, but only manifested as a slight decrease in proliferative index in response to small-bowel resection [48] . As suggested by the authors of this study, redundancy among ErbB receptors may compensate, or EGFR signalling in non-enterocytes is sufficient to sustain intestinal homeostasis. Of note, PACS-2-deficiency affects a number of ErbB ligands and hence possibly other ErbB receptors in both enterocytes and the underlying mesenchyme. This may partly explain the differences between the phenotypes of Pacs2 −/− mice and conditional intestinal Egfr knockout mice. On the basis of current literature, it is apparent that the effects of ADAM17 and EGFR deficiency on intestinal homeostasis are highly context-dependent. While there are interesting parallels, the intestinal phenotype of Pacs2 −/− mice reported here could reflect contributions from the loss of PACS-2 functions unrelated to ADAM17 and EGFR regulation. However, irrespective of the mechanisms underlying the intestinal phenotype, the reduced pEGFR levels and proliferation in Pacs2 −/− intestinal crypts are interesting observations. This reduction in proliferation was most pronounced in the small intestine as compared with the colon, likely due to higher levels of cell turnover at this site [49] . This could have important implications for intestinal cancers, which are known to arise from crypt cells in an EGFR-dependent manner [50] , [51] . Intriguingly, the genomic region encoding among other genes PACS2 is susceptible to being lost in human colorectal cancer [24] , [52] . Together, this highlights the need for further studies on the impact of PACS-2 on cancer. In summary, we report a central role for PACS-2 in ADAM17 regulation, ErbB activity, and intestinal tissue homeostasis with potential implications for cancer biology. Our findings indicate that PACS-2 regulates ADAM17 without affecting related proteases. Thus, modulating ADAM17 cell-surface availability through PACS-2 could allow for selective fine-tuning of ADAM17 activity, as a novel way of controlling ErbB signalling in cancer. Antibodies and reagents PMA and BB-94 were from Calbiochem. Geneticin, 1,10-phenanthroline monohydrate, MISSION Universal Negative Control siRNA #1, and anti-alkaline phosphatase monoclonal antibody (clone 8B6) were from Sigma-Aldrich. HALT phosphatase inhibitor cocktail was from Thermo Fisher Scientific. Complete EDTA-free inhibitor cocktail was from Roche. Interferin transfection reagent was from PolyPlus, and siGENOME non-targeting siRNA pool #2, SMARTpool PACS-2 and ADAM17 siRNAs were from Dharmacon (Thermo Scientific). We additionally used PACS-2 siRNA from Qiagen and pooled three siRNAs (PACS2_6, PACS2_7 and PACS2_9). Recombinant murine TNF-α was from Strathmann Biotec AG. PACS-2 antibody (19508-1-AP) was from Proteintech. ADAM17 (ab39162), ADAM17 (ab2051), MT1-MMP (ab38971), ADAM10 (ab1997) and pEGFR (ab40815) antibodies were from Abcam. PACS-1 antibody 17703 and PACS-2 antibody 18193 were previously described [53] , [54] . Actin (MAB1501R) and EGFR (06-847) antibodies were from Millipore. ADAM9 (AF949) and ADAM17 (MAB9301) antibodies were from R&D Systems. PACS-2-HA expression plasmid was in a pcDNA.3 backbone [40] (Invitrogen), and green fluorescent protein expression plasmid was from Clontech. Cell culture Human HT1080 fibrosarcoma cells (American Type Culture Collection (ATCC)) was cultured in Dulbecco’s Modified Eagle Medium (DMEM) with 10% fetal calf serum (FCS) at 37 °C and 5% CO 2 . Cells were transfected with cDNA constructs encoding alkaline phosphatase fused to pro-HB-EGF (AP-HB-EGF) [55] kindly provided by Professor Michael Freeman (Children’s Hospital, Boston, USA). The 10% highest-expressing cells were isolated by fluorescence-activated cell sorting and maintained by selection with 500 μg ml −1 Geneticin. HeLa and MCF-7 cells stably expressing AP-HB-EGF were kind gifts from Professors Gillian Murphy (University of Cambridge, UK) and Rosalyn Adam (Children’s Hospital, Boston, USA), respectively. AP-HB-EGF HeLa and MCF-7 cells were cultured in DMEM with 10% FCS and 800 and 600 ng ml −1 Geneticin, respectively [18] . MDA-MB-231 (ATCC) and spontaneously immortalized MEFs derived from Pacs2 −/− mice and corresponding control wild-type mice ( Pacs2 −/− MEF, control MEF) [24] were cultured in DMEM with 10% FCS. Cell lines were routinely tested for mycoplasma. Reverse transfection of siRNAs Cells were transfected with siRNAs diluted to 375 nM in Opti-MEM (Invitrogen) and Interferin transfection reagent diluted in Opti-MEM (final concentration 0.003 μl per total μl cell medium), according to the manufacturer’s instructions. Western blot Unless otherwise described, cells were washed in phosphate-buffered saline (PBS, Invitrogen) and lysed 20 min on ice in the indicated buffer. In addition to standard protease inhibitors, all lysates made to examine mature ADAM17 included 10 μM BB-94 and 10 mM 1,10-phenanthroline monohydrate in the lysis buffer to prevent ADAM17 autocleavage [10] . Equal amounts of protein were separated by reducing sodium dodecyl sulfate-polyacrylamide gel electrophoresis (SDS-PAGE) and transferred to polyvinylidene difluoride (Immobilon-P Membrane, Milipore) or nitrocellulose (Hybond ECL, GE Healthcare) membranes using standard procedures. Membranes were blocked in 5% non-fat milk or bovine serum albumin (BSA, Sigma-Aldrich), incubated overnight at 4°C with the indicated primary antibodies at dilutions of 1:500–1:1000, and subsequently with the appropriate horseradish peroxidase-conjugated secondary antibodies. Blots were visualized with LAS3000 Imager (Fujifilm) or using Hyperfilm ECL high performance chemiluminescence film (GE Healthcare). Digitally developed blots were grey-tone adjusted for figure presentation. TotalLab TL100 (TotalLab Limited) or AlphaView software (Protein Simple) was used for densitometric analysis. Shedding assay on HT1080, HeLa and MCF-7 cells AP-HB-EGF HT1080, HeLa and MCF-7 cells were reverse transfected with negative control, ADAM17 or PACS-2 siRNA in triplicate. After 72 h, HT1080 cells were washed twice with serum-free medium (SFM) and stimulated with 400 nM PMA or SFM for 30 min at 37 °C. The supernatant was transferred to 96-well plates and centrifuged. The cell layer was washed in PBS and lysed in 2 × RIPA (100 mM Tris pH 7.4, 300 mM NaCl, 0.2% SDS, 2% Triton X-100, 1% sodium deoxycholate, 2 mM EDTA, with protease inhibitor cocktail). For colorimetric quantification of shedding, the cell-conditioned medium was mixed 1:1 with a 1 mg ml −1 solution of the alkaline phosphatase substrate 4-nitrophenyl (SIGMAFAST p-Nitrophenyl phosphate Tablets, Sigma-Aldrich) in technical duplicate. After incubation at 37 °C in the dark, AP activity was quantified by measuring absorbance at 405 nm. Knockdown was verified by western blot. Forty-eight hours after transfection, AP-HB-EGF HeLa were treated with 160 nM PMA or SFM for 45 min (as described [18] ). Seventy-two hours after transfection, MCF-7 cells were stimulated with SFM, 160 nM PMA or 1 μM ionomycin for 30 min (as described [27] ). Shedding of AP-HB-EGF and knockdown efficiency were analysed as above. Flowcytometry AP-HB-EGF HT1080 cells were reverse transfected with negative control, ADAM17 or PACS-2 siRNA. After 72 h, cells were trypsinized and resuspended. After 5 min recovery, cells were washed in PBS and fixed in 4% paraformaldehyde for 20 min. Cells were subsequently washed three times in PBS, with the last wash being PBS with 1% BSA. Cells were stained for 1 h at room temperature (RT) with anti-alkaline phosphatase antibody (1:1000 dilution), washed three times, and stained with secondary Alexa Fluor 488-conjugated antibody for 1 h. Cells were washed and resuspended in PBS, and analysed using FACSCalibur (BD Biosciences). Shedding assay on control and Pacs2 −/− MEFs Control wild-type and Pacs2 −/− MEFs were reverse transfected in triplicate with AP-HB-EGF plasmid using X-tremeGENE 9 DNA transfection reagent (Roche) diluted in Opti-MEM. For rescue experiments, Pacs2 −/− MEFs were reverse transfected in triplicate with plasmid encoding AP-HB-EGF, and additionally either plasmid encoding PACS-2-HA or green fluorescent protein using Lipofectamine LTX (Invitrogen). Forty-eight hours after transfection, cells were washed twice with SFM and treated with 400 nM PMA or SFM for 1 h at 37 °C. Colorimetric quantification of shed AP-HB-EGF was performed as above. To overcome differences in transfection efficiency, the fraction of shed AP-HB-EGF was calculated as AP-HB-EGF released to the medium divided by the total amount of AP-HB-EGF in the medium and cell lysate. The ADAM17-dependent PMA-stimulated AP-HB-EGF shedding was evaluated as fold increase compared with the non-stimulated sample for each cell line. Cells were washed in PBS, lysed in 1% Triton X-100 in PBS with protease inhibitor cocktail, and western blot for PACS-2 expression performed. Quantification of endogenous HB-EGF and TGF-α release MDA-MB-231 cells were reverse transfected with negative control, ADAM17 or PACS-2 siRNA in triplicate. After 72 h, cells were washed twice in SFM and incubated for 1 h with 400 nM PMA or SFM. For TNF-α stimulation, cells were incubated with siRNA for 48 h, then starved in SFM for 24 h and stimulated with 50 ng ml −1 recombinant murine TNF-α for 5 h. In both cases, shedding of HB-EGF or TGF-α to the supernatant was assayed using Human HB-EGF or TGF-α DuoSet ELISA kits (R&D Systems), according to the manufacturer’s instructions. Cell layers were washed in PBS, lysed in 2 × RIPA and knockdown analysed by western blot. Cell-surface biotinylation assay MDA-MB-231 cells were reverse transfected with negative control, ADAM17 or PACS-2 siRNA. Seventy-two hours later, cells were washed twice in SFM and incubated with 400 nM PMA or SFM for 1 h at 37 °C. Control wild-type and Pacs2 −/− MEFs were left unstimulated. Cells were subsequently pre-incubated at 4 °C for 15 min to stop internalization. The experiment was carried out at 4 °C with cold reagents. Cells were washed twice in PBS and incubated for 30 min with 0.5 mg ml −1 non-cleavable EZ-Link Sulfo-NHS-LC-Biotin (Thermo Fisher Scientific) in PBS. Biotinylation was quenched by three washes in 100 mM glycine (AppliChem) in PBS, and additionally three PBS washes. Cells were lysed for 20 min in RIPA buffer (50 mM Tris pH 7.4; 150 mM NaCl; 0.1% SDS; 1% Triton X-100; 0.5% sodium deoxycholate; 1 mM EDTA, with protease inhibitor cocktail and 10 μM BB-94 and 10 mM 1,10-phenanthroline monohydrate). Cell lysates were cleared by centrifugation, protein concentration equalized by BCA assay and supernatants incubated with streptavidin-agarose beads (Sigma-Aldrich) for 2 h at 4 °C. Beads were washed three times in RIPA and bound proteins released by heating for 5 min at 95 °C in 2 × SDS-PAGE sample buffer. Samples were analysed by western blot. For internalization and recycling studies, MDA-MB-231 cells were siRNA transfected and biotinylated using 0.2 mg ml −1 cleavable EZ-Link Sulfo-NHS-SS-Biotin (Thermo Fisher Scientific) as described above, except cells were left unstimulated. After washing three times in 100 mM glycine in cold PBS, cells were pre-treated for 15 min with cold SFM containing 10 μM MG-132 (Sigma-Aldrich) and 10 nM Bafilomycin A1 (Sigma-Aldrich) to block protein degradation and selectively determine effects on internalization and recycling. Pre-warmed DMEM containing 10% FCS, 10 μM MG-132 and 10 nM Bafilomycin A1 was added and biotin-labelled surface proteins were allowed to internalize at 37 °C for 30 min. Internalization was stopped by transferring cells to 4 °C. Surface biotin was removed by washing three times 10 min in cold stripping buffer (50 mM reduced L-Glutathione (Sigma-Aldrich), 75 mM NaCl, 75 mM NaOH, 1% BSA and 10 mM EDTA). For recycling, cells were subsequently washed in cold PBS, pre-warmed complete medium added, and cells were incubated at 37 °C for an additional 30 min. Cells were then washed three times for 10 min with stripping buffer to remove recycled biotin-labelled proteins, washed three times in cold PBS, and lysed in RIPA. The total amount of surface biotinylation was detected by keeping a dish at 4 °C after biotin-labelling and omitting treatment with stripping buffer. To verify proper removal of surface-labelled biotin, a dish kept at 4 °C after biotin-labelling was washed with stripping buffer similarly to recycling samples, washed three times in cold PBS and lysed in RIPA. Samples were subjected to streptavidin pull-down and western blot as described. For stability studies, MDA-MB-231 cells were transfected and surface biotinylated with non-cleavable biotin as described above. Cells were then either lysed at time zero or incubated for 4 h at 37 °C in pre-warmed SFM to allow internalization and degradation of surface proteins. Cells were subsequently lysed and processed as above. ADAM17 quenched fluorescence peptide activity assay Control wild-type and Pacs2 −/− MEFs were lysed at 4 °C in RIPA containing protease inhibitor cocktail. The lysates were cleared by centrifugation, and protein concentration was equalized by BCA assay. A black Nunc Delta F96 Microwell plate was pre-coated overnight at 4 °C with a 1:100 dilution of ADAM17 antibody (ab2051, Abcam). Subsequently, the plate was washed three times in PBST (PBS with 0.05% Tween 20), and blocked in 1% BSA in PBS for 1 h at 37 °C. After washing three times in PBST, 25 μg per well of lysates were added in triplicate and incubated for 2 h at 4 °C. After washing the plate again, 5 μM of ADAM17 substrate II (5-FAM-Ser-Pro-Leu-Ala-Gln-Ala-Val-Arg-Ser-Ser-Ser-Arg-Lys(5-TAMRA)-NH 2 , ENZO Life Sciences) was added to each well for analysis of ADAM17 activity. Fluorimetric measurements with excitation at 485 nm and emission at 535 nm were made at 37 °C with an Optima FLUOSTAR plate reader (BMG Labtech), programmed for measuring every 5 min for 1 h. Deglycosylation studies Control wild-type and Pacs2 −/− MEFs were lysed in RIPA containing protease inhibitor cocktail, 10 mM 1,10-phenanthroline monohydrate and 10 μM BB-94. Lysates were denatured at 95 °C for 5 min and treated with either EndoH or PNGase F (Promega). Deglycosylation was done according to the manufacturer’s instructions and ADAM17 detected by western blot using antibody ab2051 (Abcam). Co-immunoprecipitation MDA-MB-231 cells were washed twice with SFM and treated with 400 nM PMA or SFM for 60 min at 37 °C. Cells were lysed in a buffer of 50 mM Tris pH 7.6, 150 mM NaCl, 1% NP-40, 0.25% sodium deoxycholate, standard protease inhibitors, 10 μM BB-94, 10 mM 1,10-phenanthroline monohydrate and standard phosphatase inhibitors. 5 μg of ADAM17 antibody ab39162 (Abcam) or control IgG were added to 1.16 mg total protein, and lysates were rocked overnight at 4 °C. Subsequently, lysates were incubated with Sepharose G for 2 h. After washing in lysis buffer, bound proteins were released by heating for 5 min at 100 °C in 2 × SDS-PAGE sample buffer, followed by western blot analysis. 40 μg of cell lysate was used for input controls. The reverse experiment was performed using the same protocol, but by precipitating PACS-2 with 3 μg of PACS-2 antibody 19508-1-AP (Proteintech). Control wild-type and Pacs2 −/− MEFs were subjected to the same protocol as above, except 5 μg of ADAM17 antibody ab2051 (Abcam) was added to 1.55 mg of lysate protein. Also, beads were washed in mRIPA (50 mM Tris pH 8.0, 1% NP-40, 1% deoxycholate and 150 mM NaCl). PLA Duolink II Detection Reagents Red kit with probes for mouse and rabbit reagents, based on in situ PLA technology (Olink Bioscience), was used according to the manufacturer’s instructions. MDA-MB-231 cells were reverse transfected on coverslips in duplicate with negative control, ADAM17 and PACS-2 siRNA. After 72 h, the confluent cell layer was washed twice with SFM and treated with 400 nM PMA, 40 nM PMA or SFM for 60 min at 37 °C. In parallel, one well for each siRNA transfection was lysed in 2 × RIPA and knockdown confirmed by western blot. Coverslips were washed in PBS and subsequently fixed in 10% neutral buffered formalin (Sigma-Aldrich) at RT for 20 min. Cells were permeabilised with 0.1% Triton X-100 (Sigma-Aldrich) for 15 min at RT and free aldehyde groups quenched by 15 min incubation in 0.1 M ammonium chloride, followed by three PBS washes. Blocking was performed overnight at 4 °C using 5% BSA. Primary antibodies were rabbit PACS-2 antibody (Proteintech 19508-1-AP) and mouse ADAM17 antibody (R&D Systems MAB9301). We confirmed that control IgGs did not produce signal. Antibodies were diluted 1:100 in PBS with 5% BSA, added to coverslips, and incubated for 1 h at 37 °C in a humidity chamber followed by hybridization, ligation, amplification and detection according to the manufacturer’s protocol. Nuclear staining was performed using 4′,6-diamidino-2-phenylindole (DAPI, 1 ng μl −1 , Invitrogen) before mounting coverslips in fluorescence mounting medium (Dako). Fluorescence imaging was performed using a 3D Imaging Apotome microscope with a 63 × /1.4 Plan-Apochromat water immersion objective on an inverted Zeiss Axiovert 220 Apotome system and Axiovision software (Carl Zeiss). For experiments with fluorescently labelled transferrin, MDA-MB-231 cells were seeded on coverslips in duplicate. After 48 h, the cell layer was washed twice with SFM and treated with 400 nM PMA for 60 min at 37 °C. Cells were then incubated with 10 nM Transferrin Alexa Fluor 488 (Invitrogen) together with 400 nM PMA or SFM. After 5 min, cells were rapidly transferred to 4 °C and washed in ice-cold PBS. PLA was then performed as above. Imaging was done using confocal laser-scanning microscopes LSM 510 Meta or LSM 710 (Carl Zeiss) with 63 × /1.4 oil Plan-Apochromat objectives. The fluorescence intensity of staining was measured using the program Profile, allowing the display of intensity distribution of an image along a straight line. Studies on Pacs2 −/− mice The University of Pittsburgh Division of Laboratory Animal Resources and Oregon Health & Science University Department of Comparative Medicine approved all animal studies. The Pacs2 −/− mouse line is on a C57BL/6 background [24] . Animals of both sexes were used. For immunohistochemistry, Pacs2 −/− and corresponding control wild-type mice were sacrificed at the ages indicated and ∼ 3 cm of jejunum (centred mid-way between stomach and caecum), ileum (just proximal to caecum) and colon samples were collected. Tissue samples were fixed in formalin, paraffin embedded, sectioned and processed using standard methods. Jejunum sections from 5 control and 7 Pacs2 −/− mice aged 8 weeks and colon sections from 5 control and 5 Pacs2 −/− mice aged 7–12 weeks were stained overnight with antibody against EGFR phosphorylated on Tyr1068 (Abcam ab40815, 1:200 in 10% FCS in PBS), and subsequently with Alexa Fluor 488 goat anti-rabbit antibody (Invitrogen). The staining protocol employed has been published previously and the antibody was thoroughly validated on Egfr knockout mouse tissue [38] . Nuclei were stained with DAPI. Fluorescence imaging was performed using an inverted Zeiss Axiovert 220 Apotome system with a 10 × /0.30 Plan-Neofluar or 20 × /0.75 Plan-Apochromat objective and Axiovision software (Carl Zeiss). The fluorescence intensity of pEGFR staining was measured using the confocal laser-scanning microscope LSM 510 Meta (Carl Zeiss) with a 40 × /0.14 C-Apochromat objective and the program Profile, allowing the display of intensity distribution of an image along a straight line. For each section, four images were taken at corresponding random points and the average fluorescence intensity quantified along a line averaging 193 μm across the jejunal crypts and 226 μm across colonic crypts. For Ki67 staining, jejunum samples from 5 control and 6 Pacs2 −/− mice aged 8 weeks and colon sections from 5 control and 5 Pacs2 −/− mice aged 7–12 weeks were incubated overnight with Ki67 antibody (MONX10283, Monosan, diluted 1:1000 in 10% FCS in PBS). After incubation with goat anti-mouse horseradish peroxidase-conjugated antibody (Dako), antibody binding was visualized with AEC+ Substrate-Chromogen (Dako) and sections counterstained with hematoxylin. Number and position of Ki67-positive cells were scored by manual counting of well-oriented crypts. The bottom cell of a crypt was designated as position 0, and Ki67 positivity scored at each subsequent cell up to position 30, counting both sides of each crypt individually. For each mouse, 915 crypt cells were scored, unless not enough well-oriented crypts were available. For preparation of small intestinal lysates, 7 Pacs2 −/− and 6 corresponding control wild-type mice were killed at 5 weeks of age. Ileum was isolated and lysates prepared by homogenizing crude tissue in mRIPA containing standard protease and phosphatase inhibitors. Lysates were cleared by centrifugation, protein concentration determined and were stored at −80 °C until use. The ratio of villus height to crypt depth in jejunum and ileum was quantified using 4 control and 4 Pacs2 −/− mice aged 10 weeks. More than 100 villi were counted for each genotype and segment. Colon crypt depth was measured on 5 control and 5 Pacs2 −/− mice aged 7–12 weeks. Approximately 75 colon crypts were measured for each genotype. Statistical analysis Unless otherwise stated, all data represent the average±s.e.m. of at least three independent experiments, each performed in triplicate. Data were analysed by one-way analysis of variance with Bonferroni’s or Holm-Sidak’s post hoc test for multiple comparisons or unpaired two-tailed Student’s t -test, as appropriate, using GraphPad Prism version 6.00 for Macintosh (GraphPad Software). In all cases, P <0.05 was considered statistically significant. Samples were only excluded from data if technical issues were evident. How to cite this article : Dombernowsky, S. L. et al . The sorting protein PACS-2 promotes ErbB signalling by regulating recycling of the metalloproteinase ADAM17. Nat. Commun. 6:7518 doi: 10.1038/ncomms8518 (2015).